Foxd1 is a mediator and indicator of the cell reprogramming process It remains unclear how changes in gene expression profiles that establish a pluripotent state are induced during cell reprogramming. Here we identify two forkhead box transcription factors, Foxd1 and Foxo1, as mediators of gene expression programme changes during reprogramming. Knockdown of Foxd1 or Foxo1 reduces the number of iPSCs, and the double knockdown further reduces it. Knockout of Foxd1 inhibits downstream transcriptional events, including the expression of Dax1, a component of the autoregulatory network for maintaining pluripotency. Interestingly, the expression level of Foxd1 is transiently increased in a small population of cells in the middle stage of reprogramming. The transient Foxd1 upregulation in this stage is correlated with a future cell fate as iPSCs. Fate mapping analyses further reveal that >95% of iPSC colonies are derived from the Foxd1-positive cells. Thus, Foxd1 is a mediator and indicator of successful progression of reprogramming. The ectopic expression of defined transcription factors (originally Oct4, Sox2, Klf4 and c-Myc) reprograms somatic cells into induced pluripotent stem cells (iPSCs) [1] , [2] , [3] , [4] , [5] . Fully reprogrammed iPSCs have the ability to differentiate into the three germ layers and contribute to the generation of fertile chimaeric mice. Characterization of the reprogramming process has advanced rapidly over the past few years [6] , [7] , [8] , [9] , [10] , [11] , [12] , [13] , [14] , [15] , [16] , [17] . During cell reprogramming, the global gene expression profile and the epigenetic state of somatic cells undergo dramatic changes and eventually become similar to those of embryonic stem cells (ESCs) [1] , [6] , [7] , [8] , [9] , [10] , [11] , [12] , [13] . Several reports have shown that reprogramming is a multistep process that includes accelerated cell proliferation, morphological changes of the cells, a mesenchymal-to-epithelial transition (MET) and unidentified stochastic events [12] , [13] , [14] , [15] , [16] , [17] . These events in reprogramming are currently classified into two or more phases [13] , [17] . However, many questions remain unanswered. The intermediate regulators that convey a signal from the ectopic expression of the defined transcription factors to the ESC-like gene expression profile are unknown. Molecular differences between successfully reprogrammed iPSCs and non-reprogrammed cells remain elusive. Moreover, the relationships and the sequence of the multiple events that occur during the reprogramming process are also unknown. In this study, we identify two transcription factors, Foxd1 and Foxo1, as mediators of the gene expression programme of cell reprogramming. We also identify transient upregulation of Foxd1 expression as a stage-specific marker of successful reprogramming, which may make it easier to relate the progression of the gene expression programme to other cellular events such as MET. Foxd1 and Foxo1 are predicted as mediators of reprogramming To gain insight into the hypothetical mediators and indicators of the reprogramming process, we performed time course microarray experiments. Mouse embryonic fibroblasts (MEFs) were infected with retroviruses [18] encoding either the four transcription factors (Oct4, Sox2, Klf4 and c-Myc) or GFP (control) at day 0 and sampled at day 1, 2, 3, 4, 5, 6 and 8. During the 8-day period, the expression levels of 813 probe sets were upregulated more than twofold as compared with day 0 ( Supplementary Data 1 ). Hierarchical clustering analysis showed a sequential change of the gene expression profile over time ( Fig. 1a ). The samples from day 0 and day 1 belonged to the same group as the GFP samples, and the day 2–8 samples were in another group. Additionally, the day 2–8 samples were further classified into several subgroups, and the classification was in accordance with the time points of the samples. Colonies of iPSCs were first detected around day 5 ( Supplementary Fig. 1a ), and the iPSC colonies started to express pluripotency marker genes, such as Nanog [19] , [20] and Oct4 (endogenous Oct4) [21] , around day 5–8 ( Supplementary Fig. 1b ). 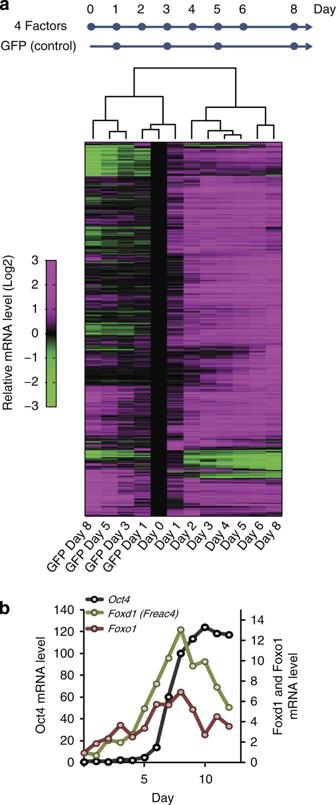Figure 1: Predicting the role of Foxd1 and Foxo1 as mediators of the gene expression programme during the reprogramming process. (a) Time course samples for microarray experiments (upper). MEFs were infected with retroviruses encoding the four transcription factors (Oct4, Sox2, Klf4 and c-Myc) or GFP at day 0. Hierarchical clustering analysis of 813 probe sets that had upregulated expression levels more than twofold as compared with day 0 (lower). (b) qRT–PCR analyses of Oct4, Foxd1 (Freac4) and Foxo1 in the reprogramming process. The increase in the expression levels of Foxd1 and Foxo1 preceded that of Oct4. Each mRNA level was normalized to the Gapdh level, and the value at day 0 was set to 1. Data are representative of five independent experiments. Figure 1: Predicting the role of Foxd1 and Foxo1 as mediators of the gene expression programme during the reprogramming process. ( a ) Time course samples for microarray experiments (upper). MEFs were infected with retroviruses encoding the four transcription factors (Oct4, Sox2, Klf4 and c-Myc) or GFP at day 0. Hierarchical clustering analysis of 813 probe sets that had upregulated expression levels more than twofold as compared with day 0 (lower). ( b ) qRT–PCR analyses of Oct4, Foxd1 (Freac4) and Foxo1 in the reprogramming process. The increase in the expression levels of Foxd1 and Foxo1 preceded that of Oct4. Each mRNA level was normalized to the Gapdh level, and the value at day 0 was set to 1. Data are representative of five independent experiments. Full size image We next attempted to identify transcription factors that regulate the gene expression profile during the reprogramming process. We used position-weight matrices of transcription factor binding sites (TFBSs) [22] , [23] to analyse the promoter sequences [24] of 411 genes that had upregulated expression levels at day 8. Among the 578 TFBSs we tested, the TFBSs for two forkhead box transcription factors, Foxd1 (also known as Freac4) and Foxo1, were the most significantly overrepresented TFBSs ( Table 1 ). Foxd1 has been shown to function in the development of the kidney and retina [25] , [26] , [27] , [28] but has never been implicated in pluripotency. Foxo1, a well-known regulator of longevity and stress response [29] , [30] , has been shown to have an essential role in maintaining the pluripotency of ESCs [31] . On the other hand, the overexpression of a dominant negative form of Foxo1 has recently been reported to increase the number of iPSC colonies [32] . Thus, the role of Foxo1 in cell reprogramming has been unclear. Table 1 Overrepresented transcription factor binding sites (TFBSs). Full size table Foxd1 and Foxo1 are transiently upregulated in reprogramming Interestingly, the expression levels of Foxd1 and Foxo1 were increased during the reprogramming process ( Fig. 1b and Supplementary Fig. 1c ), and the fold increase of Foxd1 was greater than that of Foxo1. The increase of Foxd1 and Foxo1 expression preceded that of the pluripotency marker gene, Oct4. The time required for Foxd1 and Foxo1 to reach half of the maximum expression (T 1/2 ) was 4–6 days, and the T 1/2 for Oct4 was 6–8 days ( Fig. 1b ). Furthermore, the increased expression of Foxd1 and Foxo1 was transient. The expression levels of Foxd1 and Foxo1 reached the maximum level at approximately day 8, started to decline immediately and eventually returned to near their original low levels in MEFs ( Fig. 1b ). The expression levels of Foxd1 and Foxo1 remained low in mature iPSCs and in ESCs ( Supplementary Fig. 2a ). Similar (though slower) time courses for the expression levels of Foxd1 and Foxo1 were also induced in the MEFs infected with the retroviruses for only three transcription factors (Oct4, Sox2 and Klf4) instead of four ( Supplementary Fig. 2a ). As the three-factor method [33] , [34] is more suitable for distinguishing the iPSCs from non-reprogrammed cells than the four-factor method, which produces numerous partially reprogrammed cells, we adopted the thre-factor method for the subsequent experiments. With the three-factor method, silencing of the ectopically expressed genes and the onset of the expression of the pluripotency marker genes occur around days 8–10 ( Supplementary Fig. 3 ). Note that the overexpression of any single factor of the four transcription factors did not induce Foxd1 expression nor generate iPSCs from the MEFs ( Supplementary Fig. 2b ), although the overexpression of Oct4 alone has been shown to induce Foxd1 expression in adipose tissue [35] . These results suggested a close correlation between Foxd1 expression and successful reprogramming. Knockdown of Foxd1 or Foxo1 reduces reprogramming efficiency To evaluate the significance of the transient increases in the expression of Foxd1 and Foxo1, we used lentiviruses encoding short hairpin RNAs (shRNAs) against these transcription factors. The specific shRNAs partially prevented the increase of either Foxd1 or Foxo1 expression in the reprogramming process ( Fig. 2a ). We used MEFs derived from Nanog-GFP-IRES-PuroR mice [36] , which express GFP and the puromycin resistance gene under the control of the Nanog promoter, so that we could easily assess the reprogramming efficiency. Prevention of increased Foxd1 or Foxo1 expression in the reprogramming process reduced the number of iPSC colonies ( Fig. 2b ), thereby indicating that the transient increases of Foxd1 and Foxo1 expression contributed to cell reprogramming. However, there is a possibility that the knockdown of Foxd1 or Foxo1 may affect the cell growth rate rather than the reprogramming efficiency. In particular, the MEFs treated with Foxo1 shRNA #1 often showed a reduced rate of cell proliferation. To circumvent the effect of the reduced cell number, we measured the ratio of the GFP-positive cells (that is, Nanog-positive cells) to the total cell number using FACS ( Fig. 2c and Supplementary Fig. 4 ) or measured the amount of Nanog mRNA in a fixed amount of total RNA using qRT–PCR ( Fig. 2d ). The results of both experiments showed that prevention of increased Foxd1 or Foxo1 expression reduced the ratio of iPSCs to the total number of cells, representing a reduction in the reprogramming efficiency. 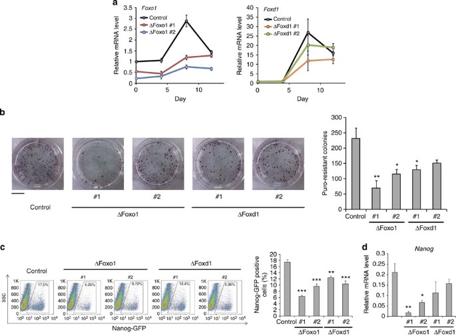Figure 2: Knockdown of either Foxd1 or Foxo1 reduces reprogramming efficiency. (a–d) Nanog-GFP-IRES-PuroR MEFs were infected with lentiviruses encoding Foxo1-specific shRNAs (ΔFoxo1 #1 or ΔFoxo1 #2), Foxd1-specific shRNAs (ΔFoxd1 #1 or ΔFoxd1 #2) or the control shRNA. After 3 days, the cells were infected with retroviruses encoding the three transcription factors (Oct4, Sox2 and Klf4). (a) Knockdown efficiency of Foxo1 (left) or Foxd1 (right) was evaluated by qRT–PCR. Data are shown as means±s.e.m. (n=3). (b) The number of puromycin-resistant colonies (that is, Nanog-positive colonies) was evaluated by alkaline phosphatase (AP) staining (left). The Nanog-GFP-IRES-PuroR MEFs were subjected to puromycin (1 μg ml−1) selection from day 14 to day 20 and then stained for AP activity at day 20. Scale bar, 10 mm. Quantification of the images (right). Data are shown as means±SEM (n=3). (c) The percentages of the GFP-positive cells (that is, Nanog-positive cells) to the total cell number were evaluated by FACS analysis at day 12 (left). The quantification of the density plots is shown (right). Data are shown as means±s.e.m. (n=4). (d) The expression levels of Nanog were evaluated by qRT–PCR at day 8. Data are shown as means±s.e.m. (n=4). (b–d) TheP-values were calculated by Dunnett’s test (***P<0.001, **P<0.01 and *P<0.05). Figure 2: Knockdown of either Foxd1 or Foxo1 reduces reprogramming efficiency. ( a – d ) Nanog-GFP-IRES-PuroR MEFs were infected with lentiviruses encoding Foxo1-specific shRNAs (ΔFoxo1 #1 or ΔFoxo1 #2), Foxd1-specific shRNAs (ΔFoxd1 #1 or ΔFoxd1 #2) or the control shRNA. After 3 days, the cells were infected with retroviruses encoding the three transcription factors (Oct4, Sox2 and Klf4). ( a ) Knockdown efficiency of Foxo1 (left) or Foxd1 (right) was evaluated by qRT–PCR. Data are shown as means±s.e.m. ( n =3). ( b ) The number of puromycin-resistant colonies (that is, Nanog-positive colonies) was evaluated by alkaline phosphatase (AP) staining (left). The Nanog-GFP-IRES-PuroR MEFs were subjected to puromycin (1 μg ml −1 ) selection from day 14 to day 20 and then stained for AP activity at day 20. Scale bar, 10 mm. Quantification of the images (right). Data are shown as means±SEM ( n =3). ( c ) The percentages of the GFP-positive cells (that is, Nanog-positive cells) to the total cell number were evaluated by FACS analysis at day 12 (left). The quantification of the density plots is shown (right). Data are shown as means±s.e.m. ( n =4). ( d ) The expression levels of Nanog were evaluated by qRT–PCR at day 8. Data are shown as means±s.e.m. ( n =4). ( b – d ) The P -values were calculated by Dunnett’s test (*** P <0.001, ** P <0.01 and * P <0.05). Full size image Foxd1 regulates reprogramming-related genes As Foxd1 has never been implicated in pluripotency, we subsequently focused on investigating the role of Foxd1 in cell reprogramming. To completely prevent the expression of Foxd1, we used MEFs derived from Foxd1 knockout mice (Foxd1-GFP-Cre mice) [27] , which express GFP-Cre instead of Foxd1 under the control of the Foxd1 promoter ( Fig. 3a ). The growth rate of the Foxd1 knockout cells ( Foxd1 −/− or Foxd1 +/− cells) was comparable to that of Foxd1 +/+ cells ( Supplementary Fig. 5 ). In agreement with the results of the knockdown experiments ( Fig. 2b–d ), the amount of Nanog mRNA ( Fig. 3b ) as well as the number of Nanog-positive iPSC colonies ( Fig. 3c ) were reduced in the Foxd1 knockout cells. These results confirmed that the expression of Foxd1 contributes to cell reprogramming. However, half as many iPSC colonies were still generated without Foxd1 ( Fig. 3c ). These Foxd1 −/− iPSCs were not significantly different from Foxd1 +/+ iPSCs in terms of the expression of the pluripotency marker genes ( Supplementary Figs 6 and 7 ), the prominent demethylation at the promoters of Oct4 and Nanog ( Supplementary Fig. 8 ), the capacity for embryoid body-mediated differentiation in vitro ( Supplementary Figs 9 and 10 ), the capacity for teratoma formation ( Supplementary Fig. 11 ) and the capacity for chimaeric mouse generation ( Supplementary Fig. 12 ). Thus, it is likely that some redundant factor should exist, which could complement the function of Foxd1 in its absence. 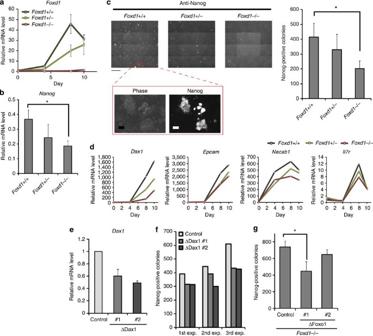Figure 3: Knockout of Foxd1 reduces reprogramming efficiency and suppresses the expression of reprogramming-related genes. (a–d) MEFs (Foxd1+/+,Foxd1+/− andFoxd1−/−) were derived from littermates of Foxd1-GFP-Cre heterozygous mating pairs. (a) The expression patterns of Foxd1 inFoxd1+/+,Foxd1+/− andFoxd1−/− MEFs were evaluated by qRT–PCR. Data are shown as means±s.e.m. (n=3). (b) The expression levels of Nanog were evaluated by qRT–PCR at day 8. Data are shown as means±s.e.m. (n=6). (c) The numbers of Nanog-positive colonies were evaluated by anti-Nanog staining at days 10–15. To create each montage image, 4 × 4 images were used (left, upper; scale bar, 4 mm). Higher magnification images of the region outlined in red are also shown (left, lower; scale bars, 200 μm); quantification of the images (right). Data are shown as means±s.e.m. (n=5). (d) The expression levels of the predicted downstream targets of Foxd1 (Dax1, Epcam, Necab1 and Il7r) were evaluated by qRT–PCR. These genes contain a Foxd1 TFBS in their promoter sequences. (e) MEFs were infected with lentiviruses encoding Dax1-specific shRNAs (ΔDax1 #1 or ΔDax1 #2) or the control shRNA. Knockdown efficiency of Dax1 was evaluated by qRT–PCR at day 8. Data are shown as means±s.e.m. (n=3). (f) The numbers of Nanog-positive colonies were evaluated by anti-Nanog staining at days 10–15. (g) TheFoxd1−/− MEFs were infected with lentiviruses encoding Foxo1-specific shRNAs (ΔFoxo1 #1 or ΔFoxo1 #2) or control shRNA. After 3 days, the cells were infected with the retroviruses encoding the three factors. The numbers of Nanog-positive colonies were evaluated by anti-Nanog staining at day 10–16 (n=3). (b,c,g) TheP-values were calculated by pairedt-test (*P<0.05). Figure 3: Knockout of Foxd1 reduces reprogramming efficiency and suppresses the expression of reprogramming-related genes. ( a – d ) MEFs ( Foxd1 +/+, Foxd1 +/− and Foxd1 −/−) were derived from littermates of Foxd1-GFP-Cre heterozygous mating pairs. ( a ) The expression patterns of Foxd1 in Foxd1 +/+, Foxd1 +/− and Foxd1 −/− MEFs were evaluated by qRT–PCR. Data are shown as means±s.e.m. ( n =3). ( b ) The expression levels of Nanog were evaluated by qRT–PCR at day 8. Data are shown as means±s.e.m. ( n =6). ( c ) The numbers of Nanog-positive colonies were evaluated by anti-Nanog staining at days 10–15. To create each montage image, 4 × 4 images were used (left, upper; scale bar, 4 mm). Higher magnification images of the region outlined in red are also shown (left, lower; scale bars, 200 μm); quantification of the images (right). Data are shown as means±s.e.m. ( n =5). ( d ) The expression levels of the predicted downstream targets of Foxd1 (Dax1, Epcam, Necab1 and Il7r) were evaluated by qRT–PCR. These genes contain a Foxd1 TFBS in their promoter sequences. ( e ) MEFs were infected with lentiviruses encoding Dax1-specific shRNAs (ΔDax1 #1 or ΔDax1 #2) or the control shRNA. Knockdown efficiency of Dax1 was evaluated by qRT–PCR at day 8. Data are shown as means±s.e.m. ( n =3). ( f ) The numbers of Nanog-positive colonies were evaluated by anti-Nanog staining at days 10–15. ( g ) The Foxd1 −/− MEFs were infected with lentiviruses encoding Foxo1-specific shRNAs (ΔFoxo1 #1 or ΔFoxo1 #2) or control shRNA. After 3 days, the cells were infected with the retroviruses encoding the three factors. The numbers of Nanog-positive colonies were evaluated by anti-Nanog staining at day 10–16 (n=3). ( b , c , g ) The P -values were calculated by paired t -test (* P <0.05). Full size image We next explored the molecular mechanism by which Foxd1 promotes iPSC generation. We measured the expression levels of the predicted downstream targets of Foxd1, which are genes containing promoters that have the Foxd1 TFBS. Some of the targets showed reduced expression levels in the Foxd1 knockout cells ( Fig. 3d ). Among them, Dax1 is an orphan nuclear receptor that is involved in the autoregulatory transcription network of ESCs [37] . The knockdown or conditional knockout of Dax1 leads to the differentiation of ESCs [38] , [39] . The expression level of Dax1 was upregulated during the reprogramming process in Foxd1 +/+ cells, but this Dax1 upregulation was completely and partially prevented in Foxd1 −/− and Foxd1 +/− cells, respectively ( Fig. 3d ). Prevention of the Dax1 upregulation in the reprogramming process by using Dax1-specific shRNAs reduced the number of Nanog-positive iPSC colonies ( Fig. 3e,f ). Epithelial cell adhesion molecule (Epcam) is a hallmark of MET that is expressed during the reprogramming process [13] . The upregulation of Epcam expression was also suppressed in the Foxd1 knockout cells ( Fig. 3d ). To systematically survey downstream targets of Foxd1 in cell reprogramming, we performed another series of microarray experiments with the Foxd1 knockout cells. Among the 813 probe sets we identified in Fig. 1a , 38 probe sets showed a ≥20% reduction in their expression levels in Foxd1 −/− cells as compared with those in Foxd1 +/+ cells at day 8 ( Supplementary Data 2 ). The Foxd1-dependent genes include pluripotency genes such as Nanog, Oct4 and Dax1. These results suggested that Foxd1 contributes to cell reprogramming by inducing expression of its downstream target genes. However, Foxd1 overexpression did not significantly change the number of iPSC colonies ( Supplementary Fig. 13 ), suggesting that there may be an optimal level of Foxd1 expression for cell reprogramming. We then examined the effect of Foxo1 downregulation in the Foxd1 knockout cells ( Supplementary Fig. 14 ). The double ablation of Foxd1 and Foxo1 further reduced the number of Nanog-positive iPSC colonies ( Fig. 3g ), suggesting that Foxd1 and Foxo1 may work redundantly during the reprogramming process. Foxd1 is an indicator of a successful reprogramming process To investigate the role of Foxd1 at the single-cell level, we used heterozygotes from the Foxd1-GFP-Cre mouse ( Foxd1 +/− mouse) as a reporter of Foxd1 expression. In agreement with the results of the qRT–PCR experiments ( Supplementary Fig. 2a , three factors), the GFP-positive cells (that is, Foxd1-positive cells) first appeared around days 6–8, reached the maximum number around day 10 and were then gradually decreased ( Fig. 4a ). Even at the maximum level (at day 10), only a small fraction (~30%) of the total cells was Foxd1-positive ( Fig. 4a ). The timing of the transient Foxd1 expression was similar to the onset of the stable expression of SSEA1 (around days 6–8), which is an early marker of the reprogramming process ( Supplementary Fig. 15a ). On the other hand, the onset of the stable expression of Nanog, which is a late marker of the reprogramming process, was much slower (around days 10–12) ( Supplementary Fig. 15b ). These results indicate that the expression of Foxd1 began to be increased in the early stage of the reprogramming process and returned to near basal level before the late stage. Next, we isolated the Foxd1-positive cells from the total cells using a cell sorter at day 8 ( Fig. 4b and Supplementary Fig. 16a ) and evaluated the reprogramming efficiencies in the later stage. More iPSC colonies were generated from the Foxd1-positive cells than from the Foxd1-negative cells ( Fig. 4c ). The putative downstream targets of Foxd1 (described in Fig. 3d ), including Dax1, showed higher expression levels in the Foxd1-positive cells than in the Foxd1-negative cells ( Supplementary Fig. 16b ). When we sorted the Foxd1-reporter cells into three fractions (that is, Foxd1++, Foxd1+ and Foxd1−) according to the expression levels of Foxd1, the Foxd1 levels were correlated well with the number of Nanog-positive iPSC colonies ( Supplementary Fig. 17 ). These results indicated that the transient increase of Foxd1 expression occurs in the middle stage of the reprogramming process and suggested that increased Foxd1 expression is an indicator of a successful progression of reprogramming. 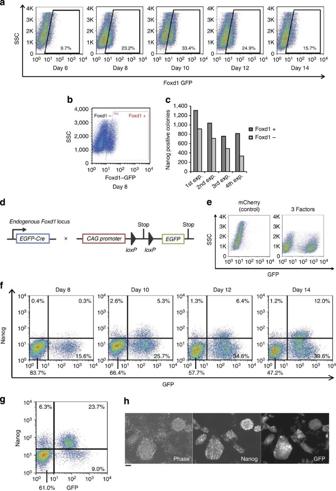Figure 4: Foxd1 is an indicator of successful progression of the reprogramming process. (a) Foxd1-GFP (+/−) MEFs were used to investigate the role of Foxd1 expression at the single-cell level. The percentages of the GFP-positive cells (that is, Foxd1-positive cells) to the total cell number were evaluated by FACS analysis at the indicated days. (b) The Foxd1-positive cells outlined in red were sorted by FACS at day 8. (c) The sorted Foxd1-positive and -negative cells were plated on new feeder layer-coated plates at day 8. The numbers of Nanog-positive colonies were evaluated by anti-Nanog staining at day 18–22. (d–h) MEFs for the fate mapping experiments were derived from mating of Foxd1-GFP-Cre mice and CAG-GFP mice. (d) Cre-mediated recombination between loxP sites results in the expression of GFP driven by the ubiquitous CAG promoter. The recombination occurs only in the cells with the expression of GFP-Cre driven by the endogenous Foxd1 promoter. (e) Cre-mediated recombination occurred at day 12 in the cells infected with the retroviruses encoding the 3 factors but not in the cells infected with the retroviruses encoding mCherry. (f) The cells were stained with Alexa Fluor 647-conjugated anti-Nanog antibodies and analysed by FACS at the indicated days. The cells first became GFP-positive (that is, the cells transiently expressed Foxd1), and later became Nanog-positive. (g) The percentages of the cells in each region to the total cell number were evaluated at day 25. The Nanog-positive cells were for the most part GFP-positive. (h) The iPSC colonies were stained with anti-Nanog antibodies and photographed at day 16. The Nanog-positive colonies were for the most part GFP-positive. Scale bar, 200 μm. Figure 4: Foxd1 is an indicator of successful progression of the reprogramming process. ( a ) Foxd1-GFP (+/−) MEFs were used to investigate the role of Foxd1 expression at the single-cell level. The percentages of the GFP-positive cells (that is, Foxd1-positive cells) to the total cell number were evaluated by FACS analysis at the indicated days. ( b ) The Foxd1-positive cells outlined in red were sorted by FACS at day 8. ( c ) The sorted Foxd1-positive and -negative cells were plated on new feeder layer-coated plates at day 8. The numbers of Nanog-positive colonies were evaluated by anti-Nanog staining at day 18–22. ( d – h ) MEFs for the fate mapping experiments were derived from mating of Foxd1-GFP-Cre mice and CAG-GFP mice. ( d ) Cre-mediated recombination between loxP sites results in the expression of GFP driven by the ubiquitous CAG promoter. The recombination occurs only in the cells with the expression of GFP-Cre driven by the endogenous Foxd1 promoter. ( e ) Cre-mediated recombination occurred at day 12 in the cells infected with the retroviruses encoding the 3 factors but not in the cells infected with the retroviruses encoding mCherry. ( f ) The cells were stained with Alexa Fluor 647-conjugated anti-Nanog antibodies and analysed by FACS at the indicated days. The cells first became GFP-positive (that is, the cells transiently expressed Foxd1), and later became Nanog-positive. ( g ) The percentages of the cells in each region to the total cell number were evaluated at day 25. The Nanog-positive cells were for the most part GFP-positive. ( h ) The iPSC colonies were stained with anti-Nanog antibodies and photographed at day 16. The Nanog-positive colonies were for the most part GFP-positive. Scale bar, 200 μm. Full size image To further evaluate the potential of Foxd1 as an indicator of the reprogramming process, we performed fate-mapping experiments. The Foxd1-GFP-Cre mice were crossed to CAG–GFP reporter mice [40] , which express GFP under the control of the CAG promoter when a loxP-flanked stop cassette is excised by Cre ( Fig. 4d,e ). Note that the GFP expression level of CAG-GFP is much higher than that of Foxd1-GFP-Cre (compare Fig. 4a,f ), indicating that the GFP fluorescence in Fig. 4e–h is attributed mostly to CAG-GFP. The GFP-positive cells (that is, the cells that had transiently expressed Foxd1 during cell reprogramming) first appeared around day 6–8, reached the maximum number (30–50%) around day 12–14 and remained high ( Fig. 4f and Supplementary Fig. 18 ). The GFP-positive cells were often SSEA1-negative ( Supplementary Fig. 19 ), suggesting that Foxd1 and SSEA1 are independently regulated. Remarkably, the GFP-positive cells frequently became Nanog-positive in the later stage ( Fig. 4g,h ). Among 316 Nanog-positive colonies, 311 colonies (95.1%) were GFP-positive ( Fig. 4h and Table 2 ). These results indicated that most of the iPSCs are derived from the Foxd1-positive cells. Table 2 The number of Foxd1-positive iPSC colonies. Full size table In this study, we have identified Foxd1 and Foxo1 as new mediators of the reprogramming process. The prevention of Foxd1 or Foxo1 expression resulted in a reduced number of iPSCs ( Figs 2 and 3 ). The role of Foxd1 in pluripotency has been revealed here for the first time. Double ablation of Foxd1 and Foxo1 further reduced the number of iPSCs ( Fig. 3g ), suggesting that multiple redundant transcription factors may contribute to cell reprogramming. The identification of these novel transcription factors should provide new insight into the molecular mechanism of cell reprogramming. The role of Foxd1 is unique in that its expression is transient unlike that of most of the reprogramming-related genes that have high expression levels in mature iPSCs or ESCs (for example, SSEA1, Nanog and Rex1) ( Fig. 1b and Supplementary Fig. 15 ). The transient increase of expression suggests that Foxd1 may be used as a stage-specific marker of the reprogramming process. The transient Foxd1 expression in this stage was correlated well with the successful generation of iPSCs in the later stage ( Fig. 4c ). More than 95% of the successful iPSC colonies were derived from the Foxd1-positive cell population ( Table 2 ). Thus, Foxd1 is a strong indicator of successful progression of the gene expression programme in cell reprogramming. As the autoregulatory network for maintaining pluripotency has been shown to consist of interlocking positive feedback loops, Foxd1 expression may trigger activation of the positive feedback loops through the induction of reprogramming-related genes such as Dax1. In fact, prevention of the induction of Dax1 resulted in a reduced number of iPSCs ( Fig. 3f ). Once the positive feedback loops are fully activated, the trigger signal of Foxd1 expression should no longer be required. One of the most interesting characteristics of cell reprogramming is that the efficiency of reprogramming is quite low (~0.1%). One explanation is that reprogramming is a multistep, stochastic process [14] , [16] , [41] . However, the stochastic events of this process are still unknown. The present study demonstrated that ~40% of the cells had shown increased Foxd1 expression in the middle stage of cell reprogramming and that most of the iPSCs are generated from the Foxd1-positive cell population in the later stage. Thus, Foxd1 expression may be one of the multiple stochastic events. It would be interesting to investigate what step(s) is stochastic during the reprogramming process from the expression of the four (or three) transcription factors to the transient expression of Foxd1. DNA constructs The pMXs vectors (pMXs-hOct4, -hSox2, -hKlf4, -hc-Myc, -GFP and -mFoxd1) were obtained from Addgene (Addgene plasmids 17217, 17218, 17219 and 17220) [1] , [18] or Cell Biolabs, Inc. pMXs-mCherry and pMXs-mFoxd1 were generated by subcloning mCherry and mFoxd1 into the pMXs vector, respectively. The shRNA sequences against Foxo1, Foxd1 and Dax1were subcloned into pENTR4-H1 (provided by Dr H. Miyoshi; RIKEN) to construct the entry vectors. The entry clones were recombined with pLenti6.3 using the Gateway technology (Invitrogen). The shRNA sequences were as follows: Control, 5′-GGCAATTACAAAATTTGATCA-3′; Foxo1_#1, 5′-GCAGCCAGGCATCTCATAACA-3′; Foxo1_#2, 5′-GCATGTTTATTGAGCGCTTGG-3′; Foxd1_#1, 5′-GAGATCTGCGAGTTCATCAGC-3′; Foxd1_#2, 5′-GCGAGATCTGCGAGTTCATCA-3′; Dax1_#1, 5′-GCAGTGCGTGAAATACATTGA-3′ and Dax1_#2, 5′-GCAGATCCTTACTGAGCACAT-3′. Cell culture protocols The MEFs, HEK293T cells (Invitrogen) and SNL 76/7 cells (ECACC) were maintained in Dulbecco’s modified Eagle’s medium (DMEM) containing 10% fetal bovine serum (FBS). The Plat-E cells (Cell Biolabs, Inc) were maintained in DMEM containing 10% FBS, puromycin (1 μg ml −1 ) and blasticidin S (10 μg ml −1 ). The cells undergoing reprogramming were cultured in a standard mouse ES medium containing 15% KnockOut Serum Replacement (KSR). Mature iPSCs (iPS-MEF-Ng-20D-17; provided by the RIKEN BRC through the Project for Realization of Regenerative Medicine and the National Bio-Resource Project of the MEXT, Japan) [36] , ESCs (CGR8) and the MEFs after cell sorting were cultured on feeder layers of mitomycin C-treated SNL76/7 cells in mouse ES medium containing 15% FBS. Mice The MEFs for the microarray and qRT–PCR analyses were derived from ICR mice. The MEFs for the knockdown experiments were derived from mating ICR mice and C57BL/6 Nanog-GFP-IRES-PuroR mice [36] (provided by the RIKEN BRC through the National Bio-Resource Project of the MEXT, Japan). The MEFs for the Foxd1 knockout experiments were derived from heterozygous mating of C57BL/6 Foxd1-GFP-Cre mice [27] . The MEFs for the fate mapping experiments were derived from the mating of Foxd1-GFP-Cre mice and C57BL/6 CAG-GFP mice [40] (provided by Dr J. Miyazaki; Osaka University). All MEFs were prepared from E13.5-E14.5 embryos. All animal studies were approved by the Animal Care and Use Committee, Graduate School of Medicine, Kyoto University. Reprogramming into iPSCs The iPSCs were induced as previously described [42] . In brief, retroviruses encoding the four transcription factors or GFP were produced in Plat-E cells. MEFs were infected with the retroviruses in DMEM containing 10% FBS (day 0) and the medium was replaced with mouse ES medium containing 15% KSR 24 h after infection. On day 2, the cells were plated onto new gelatin-coated plates. Beginning on day 3, the medium was changed every day. For the knockdown experiments, lentiviruses encoding the shRNAs against Foxd1, Foxo1 or Dax1 were produced in HEK293T cells according to the manufacturer’s protocols (Invitrogen). MEFs were infected with the lentiviruses 3 days before the infection with the retroviruses. To assess the reprogramming efficiency, the cells were stained for alkaline phosphatase (AP) activity at day 20 according to the manufacturer’s protocols (Sigma). Images for quantification were acquired with an ArrayScan VTI (Thermo Fisher Scientific). Immunocytochemistry and BrdU labelling Cells were fixed with 3.7% formaldehyde, permeabilized with 0.5% Triton X-100 and then incubated with a rabbit anti-Nanog antibody (Calbiochem, sc1000; 1/2,000). An Alexa Fluor 594-conjugated anti-rabbit antibody (Invitrogen) was used as a secondary antibody. For analysis of embryoid bodies, a rabbit anti-AFP antibody (Dako, A000829; 1/400), a goat anti-HNF3β/FoxA2 antibody (R&D, AF2400; 1/50), a mouse anti-alfa-sarcomeric actinin antibody (Sigma, A7811; 1/800), a rabbit anti GATA4 (Santa Cruz, SC-9053; 1/100), a mouse anri-Tuj1 antibody (Sigma, T8660; 1/250) and a rabbit anti-Gfap antibody (Dako, Z0334; 1/500) were used. An Alexa Fluor 488-conjugated anti-rabbit antibody (Invitrogen), an Alexa Fluor 488-conjugated anti-mouse antibody (Invitrogen) and an Alexa Fluor 488-conjugated anti-goat antibody (Invitrogen) were used as secondary antibodies. Cells labelled with 20 μM BrdU for 12 h were fixed, permeabilized and then incubated with mouse anti-BrdU antibody (BD, 347580; 1/100) and DNaseI (Takara). An Alexa Fluor 594-conjugated anti-mouse antibody (Invitrogen) was used as a secondary antibody. Images were acquired with an ArrayScan VTI, Axio Observer A1 (Carl Zeiss) or IX73 (Olympus). Immunoblotting Immunoblotting was performed by means of standard protocols. A rabbit anti-Nanog antibody (Calbiochem, sc1000; 1/1,000), a mouse anti-Oct4 antibody (Santa Cruz, sc-5279; 1/1,000), a rabbit anti-E-cadherin antibody (Cell Signaling, 24E10; 1/1,000), a rabbit anti-Foxo1 antibody (Cell Signaling, C29H4; 1/1,000) and a mouse anti-Tubulin antibody (Sigma, DM1A; 1/20,000) were used. Uncropped scans of immunoblots are shown in Supplementary Fig. 20 . Fluorescence-activated cell sorting Cells were fixed with Fixation Buffer (BD Cytofix) and permeabilized with Perm/Wash Buffer (BD Cytofix). The cells were then incubated with an Alexa Fluor 647-conjugated anti-Nanog antibody (BD, 560279; 1/1,000) or a PE-conjugated anti-SSEA1 antibody (Santa Cruz, sc21702; 1,000). The stained cells were quantified with a FACSCalibur (BD) or JSAN (Bay bioscience) and analysed with FlowJo software. Cell sorting was performed for the Foxd1-GFP fluorescence or CAG-GFP fluorescence with JSAN. qRT–PCR Total RNA was extracted with an RNeasy kit (Qiagen) and reverse transcribed with a QuantiTect Reverse Transcription Kit (Qiagen). PCR was performed with a LightCycler 480 II (Roche). The measured value was normalized to glyceraldehyde-3-phosphate dehydrogenase (Gapdh). The primers used for the PCR analysis were as follows: Gapdh, 5′-TGCAGTGGCAAAGTGGAGATT-3′ and 5′-CCTTGACTGTGCCGTTGAATT-3′; Foxo1, 5′-AAGAGCGTGCCCTACTTCAA-3′ and 5′-TGCTGTGAAGGGACAGATTG-3′; Foxd1, 5′-TACTCGTACATCGCGCTCAT-3′ and 5′-CTGCTGATGAACTCGCAGAT-3′; Nanog, 5′-AAGCGGTGGCAGAAAAAC-3′ and 5′-GCAATGGATGCTGGGATACT-3′; mOct4, 5′-TCTGTTCCCGTCACTGCTC-3′ and 5′-ATTTAACCCCAAAGCTCCAG-3′; mSox2, 5′-ATGGCCCAGCACTACCAG-3′ and 5′-CCTCCCAATTCCCTTGTATC-3′; mKlf4, 5′-CCACCTTGCCTTACACATGA-3′ and 5′-TGGGAAGACAGTGTGAAAGG-3′; hOct4, 5′-GCTCCTGAAGCAGAAGAGGA-3′ and 5′-AGATGGTCGTTTGGCTGAAT-3′; hSox2, 5′-AACCCCAAGATGCACAACTC-3′ and 5′-TCTCCGTCTCCGACAAAAGT-3′; hKlf4, 5′-GGAGAAGACACTGCGTCAAG-3′ and 5′-AGTCGCTTCATGTGGGAGA-3′; Gfp, 5′-GACGACGGCAACTACAAGAC-3′ and 5′-TCGGCCATGATATAGACGTT -3′; Dax1, 5′-TATCTGAAAGGGACCGTGCT-3′ and 5′-TCTCCACTGAAGACCCTCAA-3′; Epcam, 5′-GGCAACAAGTTGCTCTCTGA-3′ and 5′-TTCATCGCCAAGCATTTAGA-3′; Necab1, 5′-GGAGAACAGCAGTGTGTGGA-3′ and 5′-TGCTTCTTTGGAACGTCTTG-3′; Il7r, 5′-TGGAAGTGGATGGAAGTCAA-3′ and 5′-ACTCGTAAAAGAGCCCCACA-3′; Afp, 5′-TCCAGAAGGAAGAGTGGACAA-3′ and 5′-GCAGACTAGGAGAAGAGAAATAGTTGA-3′; Gata6, 5′-CCCTCATCAAGCCACAGAA-3′ and 5′-GGTTGTGGTGTGACAGTTGG-3′; Gata4, 5′-TCTCACTATGGGCACAGCAG-3′ and 5′-GCGATGTCTGAGTGACAGGA-3′; SM-actin, 5′-CTGACAGAGGCACCACTGAA-3′ and 5′-AGAGGCATAGAGGGACAGCA-3′; Cdx2, 5′-CAAGGACGTGAGCATGTATCC-3′ and 5′-GTAACCACCGTAGTCCGGGTA-3′; and Nestin, 5′-CCCTGAAGTCGAGGAGCTG-3′ and 5′-CTGCTGCACCTCTAAGCGA-3′. Promoter methylation analysis Genomic DNA of MEFs and iPSCs were isolated and bisulphite sequencing was performed with the EZ DNA Methylation-Direct Kit (Zymo Research). The promoter regions of Nanog and Oct4 were amplified with nested PCR primer sets. The amplified PCR products were ligated into pCRII-TOPO (Invitrogen) and sequenced with M13 forward and reverse primers. The primers used for the PCR were as follows: Nanog promoter 1st, 5′-GGATGTTTTTAGATTAGAGGATGTTTTTTA-3′ and 5′-ACCAAAAAAACCCACACTCATATCAATATA-3′; Nanog promoter 2nd, 5′-AATGTTTATGGTGGATTTTGTAGGT-3′ and 5′-CCCACACTCATATCAATATAATAAC-3′; Oct4 promoter 1st, 5′-TTGTTTTGTTTTGGTTTTGGATATGGGTTG-3′ and 5′-CCCAATCCCACCCTCTAACCTTAAC-3′; and Oct4 promoter 2nd, 5′-ATGGGTTGAAATATTGGGTTTATTTA-3′ and 5′-CCACCCTCTAACCTTAACCTCTAAC-3′. Teratoma formation The iPSCs were isolated and suspended at 1 × 10 7 cells per ml in KSR medium. The cell suspension (100 μl) was mixed with 100 μl Matrigel (BD, 356234) and injected subcutaneously into BALB/c-nu/nu mice (10 weeks old, female). Five weeks later, teratomas were surgically dissected, fixed in PBS containing 4% paraformaldehyde and analysed. Paraffin-embedded teratomas were stained with hematoxylin and eosin. Embryoid body-mediated in vitro differentiation The iPSCs were isolated and suspended at 7.5 × 10 3 cells per ml in ES medium containing 15% FCS. The cell suspension (100 μl) was transferred into Ultra Low Attachment 96-plates and cultured for 5 days. The aggregated cells were plated onto gelatine-coated dishes and cultured for another 10 days. The cells were analysed by immunocytochemistry and qRT–PCR. Chimaeric mouse generation The iPSCs (C57BL/6) were injected into host blastocysts (ICR) and transferred into pseudopregnant females (ICR). Chimaerism was ascertained after birth by the coat colour. Microarray analysis Two biological replicates were prepared for microarray samples. Total RNA was extracted with an RNeasy kit (Qiagen). The target preparation, hybridization to a Mouse Gene 1.0 ST Array, and scanning were performed according to the manufacturer’s protocols (Affymetrix). The probe set signals were calculated with the robust multi-array average (RMA) algorithm of GeneSpring software (Agilent). The annotation is based on na32 (mm9). Statistical analysis was performed by one-way analysis of variance (ANOVA) with a Benjamini and Hochberg false discovery rate (BH-FDR=0.1). The probe sets that had low signals (<100) in all samples were excluded from the analysis. Hierarchical clustering was performed with the Matlab software (MathWorks). Promoter analysis The 411 genes (629 probe sets) that had upregulated expression levels more than twofold at day 8 as compared with day 0 were used for promoter analysis. The promoter sequences (1.2 kb) were obtained from DBTSS [24] . The sequences were scanned with MATCH [22] using 578 position–weight matrices of vertebrate TFBSs [23] (cutoff=minSUM). For each TFBS, the ratio of genes that had promoter sequences containing the TFBS in the 411 upregulated genes was compared with the ratios in all 13,175 genes with a Fisher’s exact test of the R software. Accession codes: Microarray data were deposited in the NCBI GEO database with accession numbers GSE38509 and GSE51179 . How to cite this article: Koga, M. et al. Foxd1 is a mediator and indicator of the cell reprogramming process. Nat. Commun. 5:3197 doi: 10.1038/ncomms4197 (2014).